Photochemical reflectance index as an indirect estimator of foliar isoprenoid emissions at the ecosystem level Terrestrial plants re-emit around 1–2% of the carbon they fix as isoprene and monoterpenes. These emissions have major roles in the ecological relationships among living organisms and in atmospheric chemistry and climate, and yet their actual quantification at the ecosystem level in different regions is far from being resolved with available models and field measurements. Here we provide evidence that a simple remote sensing index, the photochemical reflectance index, which is indicative of light use efficiency, is a good indirect estimator of foliar isoprenoid emissions and can therefore be used to sense them remotely. These results open new perspectives for the potential use of remote sensing techniques to track isoprenoid emissions from vegetation at larger scales. On the other hand, our study shows the potential of this photochemical reflectance index technique to validate the availability of photosynthetic reducing power as a factor involved in isoprenoid production. Isoprene and monoterpenes (a diverse group of molecules made up of two isoprene units) are biogenic volatile organic compounds (BVOC) emitted from vegetation and are of great importance in plant biology and ecology as well as in atmospheric chemistry and climate [1] , [2] . Total BVOC emissions are estimated to be around 1 Pg C a −1 , of which isoprene and monoterpenes represent more than half [3] , [4] . These emissions of volatile isoprenoids have a significant effect on the atmospheric content of greenhouse gases and pollutants and secondary organic aerosols [5] , [6] , and thus also on climate [1] , [2] , [7] . Isoprenoid emissions at the foliar, canopy and regional level are generally estimated using models based on leaf emission capacities ( E c ), which are emission rates measured at the leaf level under standard light and temperature conditions [8] , [9] , [10] . Temporal and spatial variations in emissions are derived by modifying E c using empirical equations that describe the observed short-term controls based on temperature and light, and long-term controls based on antecedent weather conditions and environmental and biotic stresses [3] , [8] , [9] , [10] . E c were initially considered to be species-specific constants. There is now multiple evidence showing that E c values are very variable and acclimate seasonally and over environmental gradients [9] , [10] . These models are now increasing in complexity in order to manage these variations in E c empirically [11] ; they use empirical functions to describe the relationships between emission rates, environmental variables and serial multipliers based on single-factor relationships in order to account for co-variations of environmental variables that improve the estimates. However, these estimates remain unsatisfactory [11] . Current efforts are now being made to base the modelling on a fundamental understanding of plant biology [11] , [12] , nevertheless, uncertainty remains high [3] , [11] , [12] . For example, MEGAN isoprene flux estimates were within a factor of 2 above-canopy fluxes measured over a growing season in northern Michigan [3] . Emissions and BVOC budgets can also be estimated by inverse modelling based on atmospheric concentrations [13] , [14] , but the actual ground and aircraft measuring of atmospheric concentrations remains both laborious and sporadic. In addition to estimates based on modelling, isoprenoid emissions can be directly measured at the canopy level by applying eddy-covariance techniques [15] , [16] , [17] ; this is currently the only direct way to measure BVOC flux of whole ecosystems with a high temporal resolution. However, these measurements are scarce and limited to a few small sites. Eddy-covariance techniques applied from towers can be effectively used to measure only a single ‘point’ over a flat and uniform terrain, usually in the order of a few hundred or thousand square metres. When applied from aircraft, eddy-covariance techniques can be used to measure several sites [18] , but studies are few in number and temporally very limited. The spatial and temporal extension of isoprenoid flux assessment can be provided by the application of remote sensing techniques. Indirect approaches exist for the remote sensing of isoprenoid emissions through the detection of one of its oxidation products: formaldehyde (for example refs 12 , 19 ). This approach relies on assumptions associated with the oxidant chemistry relating isoprenoids to formaldehyde that are subject to significant uncertainties [19] . Isoprenoid emissions can also be remotely sensed indirectly through detectable changes in carotenoid concentrations that are related to isoprenoid emissions [20] . Detecting BVOC exchange using remote sensing techniques is, however, a very challenging goal, and one that is far from being accomplished. Here, our aim is to determine a simple remote sensing approach that extends our ability to assess isoprenoid fluxes in space and time. We assume a negative relationship between light use efficiency (LUE; here calculated as the ratio between measured net photosynthetic rates and incident photosynthetic photon flux density (PPFD) in mol CO 2 mol per photons) and isoprenoid emissions as a result of a higher availability of photosynthetic reducing power and substrate for isoprenoid production under lower LUEs [12] , [21] , [22] . The photochemical reflectance index (PRI), which is calculated as (R531−R570)/(R531+R570), where Rn is the reflectance of the leaf at n nm is a good estimator of LUE at the leaf, canopy and ecosystem levels [23] , [24] , [25] , [26] , [27] . We, therefore, hypothesize that PRI would also be useful as an estimator of isoprenoid emissions. We test our hypothesis on saplings of a deciduous species, Populus nigra L., an isoprene emitter, and an evergreen species, Quercus ilex L., which is mostly a monoterpene emitter. We calculate light-response curves for isoprenoid emissions from 0–2500 μmol m −2 s −1 in leaves of saplings growing under well-irrigated conditions, under drought conditions and under conditions of senescence, and in all cases compare growth in full sun with shade, that is, we generate a wide range of LUEs to test our hypothesis. The results provide evidence that PRI is a good indirect estimator of foliar isoprenoid emissions and can therefore be used to sense them remotely. The results also show the potential of this PRI technique to validate the availability of photosynthetic reducing power as a factor involved in isoprenoid production. Relationships of isoprenoid emissions with LUE Isoprenoid emissions were always negatively related to LUE both for isoprene in P. nigra and for monoterpenes in Q. ilex in response to irradiance and in each environment of drought, senescence and light growth ( Fig. 1 ). Under each experimental condition and for individual leaves, LUE accounted for up to 90% of the variance in isoprene and monoterpene emissions. LUE explained 73 and 72% of the total variance in isoprene and monoterpene emission rates expressed as a percentage of the maximum emission rate measured per plant and growth condition, when the whole data set for all cases and conditions was considered ( Fig. 2 ). LUE explained 40 and 42% of the total variance when absolute values of isoprene and monoterpene emission rates were considered ( Fig. 3 ). All these relationships still held when considering only the light-saturated conditions with constant net photosynthetic rates and changing electron transport rates (above 250 μmol m −2 s −1 , Fig. 2 , Fig. 4 ). 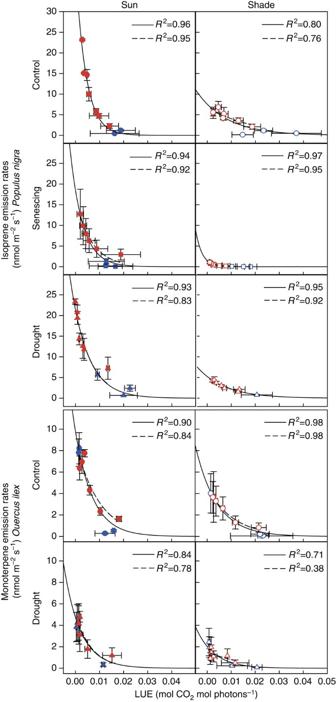Figure 1: Relationships between foliar isoprenoid emissions and LUE for each growing condition. Isoprene emission rates ofPopulus nigraand monoterpene emission rates ofQuercus ilexas a function of light use efficiency (LUE) in control, foliar senescing and droughted plants grown in sunny (closed symbols) and shaded (open symbols) conditions. The red symbols and the dashed lines represent light-saturated conditions for photosynthesis (PAR above 250 μmol m−2s−1). The blue symbols represent values for PAR below 250 μmol m−2s−1, that is, with not saturated photosynthetic rates (Fig. 4). The continuous line represents the whole data set. The error bars are±s.e. (n=3 plants). Figure 1: Relationships between foliar isoprenoid emissions and LUE for each growing condition. Isoprene emission rates of Populus nigra and monoterpene emission rates of Quercus ilex as a function of light use efficiency (LUE) in control, foliar senescing and droughted plants grown in sunny (closed symbols) and shaded (open symbols) conditions. The red symbols and the dashed lines represent light-saturated conditions for photosynthesis (PAR above 250 μmol m −2 s −1 ). The blue symbols represent values for PAR below 250 μmol m −2 s −1 , that is, with not saturated photosynthetic rates ( Fig. 4 ). The continuous line represents the whole data set. The error bars are±s.e. ( n =3 plants). 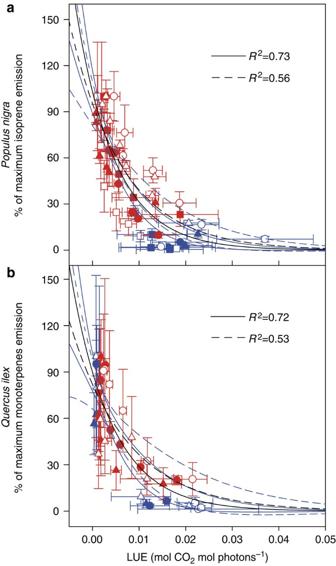Figure 2: Relationship between isoprenoid emissions and LUE for all growing conditions. Isoprene emission rates ofPopulus nigra(a) and monoterpene emission rates ofQuercus ilex(b) (relative to the maximum for each plant) as a function of light use efficiency (LUE) considering control, foliar senescing and droughted plants grown in sunny (closed symbols) and shaded (open symbols) conditions altogether. The red symbols and the dashed black line represent light-saturated conditions for photosynthesis (PAR above 250 μmol m−2s−1). The blue symbols represent values for PAR below 250 μmol m−2s−1, that is, with not saturated photosynthetic rates (Fig. 4). The continuous black line represents the whole data set. The error bars of the symbols are±s.e. (n=3 plants). SEE, standard error of estimate. 95% Confidence intervals are plotted for both relationships (continuous blue lines for whole data set and dashed blue lines for light-saturated conditions for photosynthesis). For the whole data set:y=aexp (-bx) wherea=103±7,b=119±15, SEE 17. For the data set on light-saturated conditions:y=aexp (-bx) wherea=95±7,b=89±16, SEE 18. For the whole data set on monoterpene emissions:y=aexp (-bx) where a =90±6, b=114±21, SEE 18. For the data set on light-saturated conditions:y=aexp (-bx) where a=82±8, b=81±23, SEE 18.5. Full size image Figure 2: Relationship between isoprenoid emissions and LUE for all growing conditions. Isoprene emission rates of Populus nigra ( a ) and monoterpene emission rates of Quercus ilex ( b ) (relative to the maximum for each plant) as a function of light use efficiency (LUE) considering control, foliar senescing and droughted plants grown in sunny (closed symbols) and shaded (open symbols) conditions altogether. The red symbols and the dashed black line represent light-saturated conditions for photosynthesis (PAR above 250 μmol m −2 s −1 ). The blue symbols represent values for PAR below 250 μmol m −2 s −1 , that is, with not saturated photosynthetic rates ( Fig. 4 ). The continuous black line represents the whole data set. The error bars of the symbols are±s.e. ( n =3 plants). SEE, standard error of estimate. 95% Confidence intervals are plotted for both relationships (continuous blue lines for whole data set and dashed blue lines for light-saturated conditions for photosynthesis). For the whole data set: y = a exp (- bx ) where a =103±7, b =119±15, SEE 17. For the data set on light-saturated conditions: y = a exp (- bx ) where a =95±7, b =89±16, SEE 18. For the whole data set on monoterpene emissions: y = a exp (- bx ) where a =90±6, b=114±21, SEE 18. For the data set on light-saturated conditions: y = a exp (- bx ) where a=82±8, b=81±23, SEE 18.5. 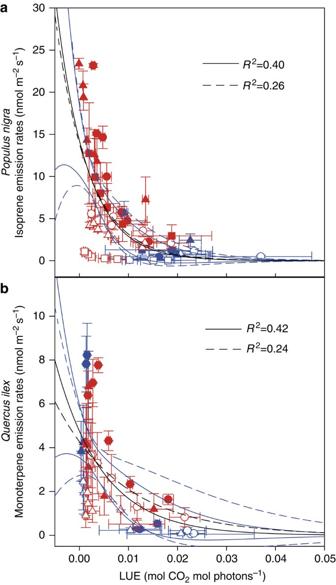Figure 3: Relationship between isoprenoid emissions and LUE for all growing conditions. Isoprene emission rates ofPopulus nigra(a) and monoterpene emission rates ofQuercus ilex(b) (expressed in absolute values) as a function of light use efficiency (LUE) considering control, foliar senescing and droughted plants grown in sunny (closed symbols) and shaded (open symbols) conditions altogether. The red symbols and the dashed black line represent light-saturated conditions for photosynthesis (PAR above 250 μmol m−2s−1). The blue symbols represent values for PAR below 250 μmol m−2s−1, that is, with not saturated photosynthetic rates (Fig. 4). The continuous black line represents the whole data set. The error bars of the symbols are±s.e. (n=3 plants). SEE, standard error of estimate. 95% Confidence intervals are plotted for both relationships (continuous blue lines for whole data set and dashed blue lines for light-saturated conditions for photosynthesis). For the whole data set:y=aexp (-bx) where a=14±2, b=160±41, SEE 4.8. For the data set on light-saturated conditions:y=aexp (-bx) wherea=14±2.5,b=148±52, SEE 5.6. For the whole data set on monoterpene emissions:y=aexp (-bx) where a=4.75±0.6, b=104±35, SEE 1.8. For the data set on light-saturated conditions:y=aexp (-bx) wherea=4.3±0.7,b=71±38, SEE 1.8. Full size image Figure 3: Relationship between isoprenoid emissions and LUE for all growing conditions. Isoprene emission rates of Populus nigra ( a ) and monoterpene emission rates of Quercus ilex ( b ) (expressed in absolute values) as a function of light use efficiency (LUE) considering control, foliar senescing and droughted plants grown in sunny (closed symbols) and shaded (open symbols) conditions altogether. The red symbols and the dashed black line represent light-saturated conditions for photosynthesis (PAR above 250 μmol m −2 s −1 ). The blue symbols represent values for PAR below 250 μmol m −2 s −1 , that is, with not saturated photosynthetic rates ( Fig. 4 ). The continuous black line represents the whole data set. The error bars of the symbols are±s.e. ( n =3 plants). SEE, standard error of estimate. 95% Confidence intervals are plotted for both relationships (continuous blue lines for whole data set and dashed blue lines for light-saturated conditions for photosynthesis). For the whole data set: y = a exp (- bx ) where a=14±2, b=160±41, SEE 4.8. For the data set on light-saturated conditions: y = a exp (- bx ) where a =14±2.5, b =148±52, SEE 5.6. For the whole data set on monoterpene emissions: y = a exp (- bx ) where a=4.75±0.6, b=104±35, SEE 1.8. For the data set on light-saturated conditions: y = a exp (- bx ) where a =4.3±0.7, b =71±38, SEE 1.8. 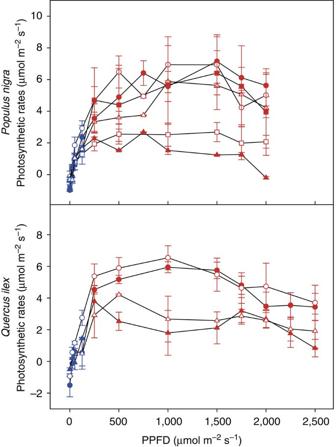Figure 4: Light-response curves of net photosynthetic rates ofPopulus nigraandQuercus ilex. Data shown for net photosynthetic rates in control (circles), foliar senescing (squares) and droughted (triangles) plants grown in sunny (closed symbols) and shaded conditions (open symbols). The error bars are±s.e. (n=3 plants). PPFD, photosynthetic photon flux density. The figure shows saturation of net photosynthetic rates at PPFDs above 250 μmol m−2s−1The red symbols represent light-saturated conditions for photosynthesis (PAR above 250 μmol m−2s−1). The blue symbols represent values for PAR below 250 μmol m−2s−1, that is, with non-saturated photosynthetic rates. Full size image Figure 4: Light-response curves of net photosynthetic rates of Populus nigra and Quercus ilex. Data shown for net photosynthetic rates in control (circles), foliar senescing (squares) and droughted (triangles) plants grown in sunny (closed symbols) and shaded conditions (open symbols). The error bars are±s.e. ( n =3 plants). PPFD, photosynthetic photon flux density. The figure shows saturation of net photosynthetic rates at PPFDs above 250 μmol m −2 s −1 The red symbols represent light-saturated conditions for photosynthesis (PAR above 250 μmol m −2 s −1 ). The blue symbols represent values for PAR below 250 μmol m −2 s −1 , that is, with non-saturated photosynthetic rates. Full size image Relationships of isoprenoid emissions with PRI When we tested PRI thereafter, with the reflectance index used as a proxy for LUE in order to assess isoprene and monoterpene emission rates remotely, we found that, in effect, isoprenoid emissions were negatively related to PRI both for isoprene in P. nigra and for monoterpenes in Q. ilex in response to irradiance and to each particular drought, senescence and light growth environment ( Fig. 5 ). PRI explained more than 90% of the variance in isoprene and monoterpene emission rates for most growth conditions and plants when considered separately and in sunny conditions ( Fig. 5 ), and 65% of the variance in isoprene emission rates and 57% of the variance in monoterpene emission rates when considering the whole set of data under all the different drought, light, senescence and sun–shade conditions ( Fig. 6 ). It still explained 58 and 47% of the respective variances in isoprene and monoterpene emission rates, respectively, when considering only the light-saturated conditions (above 250 μmol m −2 s −1 , Fig. 6 ). 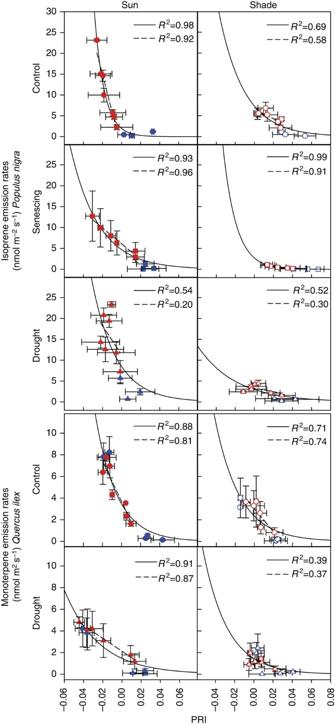Figure 5: The relationships between foliar isoprenoid emissions and PRI for each growing condition. Isoprene emission rates ofPopulus nigraand monoterpene emission rates ofQuercus ilexas a function of photochemical reflectance index (PRI) in control, foliar senescing and droughted plants grown in sunny (closed symbols) and shaded (open symbols) conditions. The red symbols and the dashed lines represent light-saturated conditions for photosynthesis (PAR above 250 μmol m−2s−1). The blue symbols represent values for PAR below 250 μmol m−2s−1, that is, with not saturated photosynthetic rates (Fig. 4). The continuous lines represent the whole data set. The error bars are±s.e. (n=3 plants). Figure 5: The relationships between foliar isoprenoid emissions and PRI for each growing condition. Isoprene emission rates of Populus nigra and monoterpene emission rates of Quercus ilex as a function of photochemical reflectance index (PRI) in control, foliar senescing and droughted plants grown in sunny (closed symbols) and shaded (open symbols) conditions. The red symbols and the dashed lines represent light-saturated conditions for photosynthesis (PAR above 250 μmol m −2 s −1 ). The blue symbols represent values for PAR below 250 μmol m −2 s −1 , that is, with not saturated photosynthetic rates ( Fig. 4 ). The continuous lines represent the whole data set. The error bars are±s.e. ( n =3 plants). 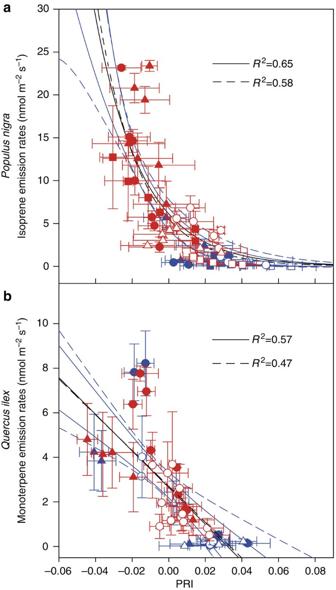Figure 6: Relationship between foliar isoprenoid emissions and PRI for all growing conditions. Isoprene emission rates ofPopulus nigra(a) and monoterpene emission rates ofQuercus ilex(b) as a function of photochemical reflectance index (PRI) considering control, foliar senescing and droughted plants grown in sunny (closed symbols) and shaded (open symbols) conditions altogether. The red symbols and the dashed black line represent light-saturated conditions for photosynthesis (PAR above 250 μmol m−2s−1). The blue symbols represent values for PAR below 250 μmol m−2s−1, that is, with not saturated photosynthetic rates (Fig. 4). The continuous black line represents the whole data set. The error bars of the symbols are±s.e. (n=3 plants). SEE, standard error of estimate. 95% Confidence intervals are plotted for both relationships (continuous blue lines for whole data set and dashed blue lines for light-saturated conditions for photosynthesis). For the whole data set on isoprene emissions:y=aexp (-bx) wherea=5.5±0.6,b=43.6±5.6, SEE 3.6. For the data set on light-saturated conditions:y=aexp (-bx) wherea=6.1±0.8,b=39±7, SEE 4.2. For the whole data set on monoterpene emissions:y=aexp (-bx) wherea=2.6±0.2,b=−82±11, SEE 1.5. For the data set on light-saturated conditions:y=aexp (-bx) wherea=2.7±0.3,b=−80±18, SEE 1.5. Full size image Figure 6: Relationship between foliar isoprenoid emissions and PRI for all growing conditions. Isoprene emission rates of Populus nigra ( a ) and monoterpene emission rates of Quercus ilex ( b ) as a function of photochemical reflectance index (PRI) considering control, foliar senescing and droughted plants grown in sunny (closed symbols) and shaded (open symbols) conditions altogether. The red symbols and the dashed black line represent light-saturated conditions for photosynthesis (PAR above 250 μmol m −2 s −1 ). The blue symbols represent values for PAR below 250 μmol m −2 s −1 , that is, with not saturated photosynthetic rates ( Fig. 4 ). The continuous black line represents the whole data set. The error bars of the symbols are±s.e. ( n =3 plants). SEE, standard error of estimate. 95% Confidence intervals are plotted for both relationships (continuous blue lines for whole data set and dashed blue lines for light-saturated conditions for photosynthesis). For the whole data set on isoprene emissions: y = a exp (- bx ) where a =5.5±0.6, b =43.6±5.6, SEE 3.6. For the data set on light-saturated conditions: y = a exp (- bx ) where a =6.1±0.8, b =39±7, SEE 4.2. For the whole data set on monoterpene emissions: y = a exp (- bx ) where a =2.6±0.2, b =−82±11, SEE 1.5. For the data set on light-saturated conditions: y = a exp (- bx ) where a =2.7±0.3, b =−80±18, SEE 1.5. Full size image We randomly selected two out of the three replicates for each growth condition and used them as the training set for estimating isoprenoid emission rates from PRI. The estimated values were then tested against the values of the remaining randomly selected third set of replicates. This procedure was repeated 1,000 times. We determined there to be a strong fit of the observed emission rates compared with those predicted by the PRI empirical model (RMSE of 2.69 nmol m −2 s −1 for isoprene emissions and 1.54 nmol m −2 s −1 for monoterpene emissions; Fig. 7 ). 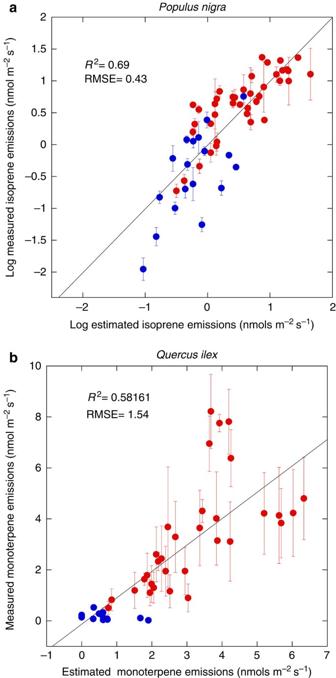Figure 7: Observed versus predicted isoprenoid emission rates. Empirical relationships with PRI are used to plot observed and predicted isoprenoid emission rates on log (a) and normal (b) scales. The error bars are±s.e. (n=3 plants). The plotted line is the 1:1 line. The red symbols correspond to light-saturated conditions for photosynthesis (PAR above 250 μmol m−2s−1). The blue symbols represent values for PAR below 250 μmol m−2s−1, that is, with not saturated photosynthetic rates (Fig. 4). Figure 7: Observed versus predicted isoprenoid emission rates. Empirical relationships with PRI are used to plot observed and predicted isoprenoid emission rates on log ( a ) and normal ( b ) scales. The error bars are±s.e. ( n =3 plants). The plotted line is the 1:1 line. The red symbols correspond to light-saturated conditions for photosynthesis (PAR above 250 μmol m −2 s −1 ). The blue symbols represent values for PAR below 250 μmol m −2 s −1 , that is, with not saturated photosynthetic rates ( Fig. 4 ). Full size image We also found that PRI explained significant variance of the residuals of the estimations of standard emission models such as MEGAN [3] both for isoprene and monoterpene emissions ( Fig. 8 ), and that PRI, together with basal emission factors, was a similar predictor for isoprenoids as these standard emission models ( Fig. 9 ). Finally, better predictions for isoprene emissions and similar or slightly better predictions for monoterpene emissions were obtained by complementing MEGAN algorithms with PRI ( Fig. 9 ). 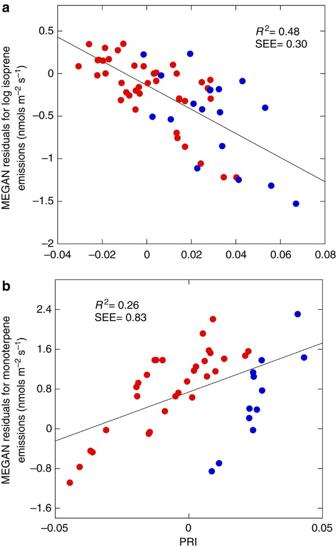Figure 8: Relationships of the residuals of MEGAN-estimated emissions with PRI. Emission rates were expressed as log nmol m−2s−1for isoprene, and as nmol m−2s−1for monoterpenes. No error bars for observations are plotted here; they are shown inFig. 7. The plotted line is the 1:1 line. The red symbols correspond to light-saturated conditions for photosynthesis (PAR above 250 μmol m−2s−1). The blue symbols represent values for PAR below 250 μmol m−2s−1, that is, with not saturated photosynthetic rates (Fig. 4). Figure 8: Relationships of the residuals of MEGAN-estimated emissions with PRI. Emission rates were expressed as log nmol m −2 s −1 for isoprene, and as nmol m −2 s −1 for monoterpenes. No error bars for observations are plotted here; they are shown in Fig. 7 . The plotted line is the 1:1 line. The red symbols correspond to light-saturated conditions for photosynthesis (PAR above 250 μmol m −2 s −1 ). The blue symbols represent values for PAR below 250 μmol m −2 s −1 , that is, with not saturated photosynthetic rates ( Fig. 4 ). 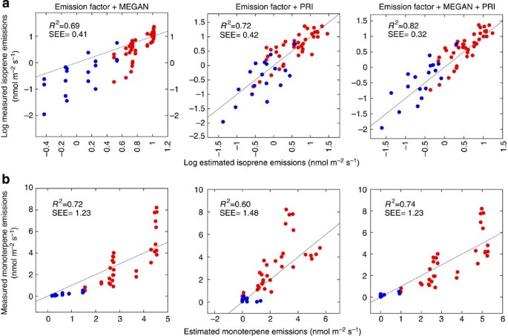Figure 9: Adding PRI to the estimation of isoprenoid emissions. Measured versus estimated isoprenoid emissions using MEGAN model, PRI and MEGAN+PRI to scale the basal emission factors. No error bars for observations are plotted here; they are shown inFig. 7. The plotted line is the 1:1 line. The red symbols correspond to light-saturated conditions for photosynthesis (PAR above 250 μmol m−2s−1). The blue symbols represent values for PAR below 250 μmol m−2s−1, i.e., with not saturated photosynthetic rates (Fig. 4). Full size image Figure 9: Adding PRI to the estimation of isoprenoid emissions. Measured versus estimated isoprenoid emissions using MEGAN model, PRI and MEGAN+PRI to scale the basal emission factors. No error bars for observations are plotted here; they are shown in Fig. 7 . The plotted line is the 1:1 line. The red symbols correspond to light-saturated conditions for photosynthesis (PAR above 250 μmol m −2 s −1 ). The blue symbols represent values for PAR below 250 μmol m −2 s −1 , i.e., with not saturated photosynthetic rates ( Fig. 4 ). Full size image The inverse relationships found between isoprenoid emissions and PRI, and therefore the significant predictive value of the latter (RMSE was 2.69 nmol m −2 s −1 for the estimation of emission rates of isoprene ranging from 0 and 25 nmol m −2 s −1 in P. nigra and 1.54 nmol m −2 s −1 for the estimation of the emission rates of monoterpenes ranging from 0 to 10 nmol m −2 s −1 in Q. ilex ; Fig. 5 ), fitted well with our hypothesis that isoprenoid emissions could be remotely sensed using PRI at the leaf level. This remote sensing capacity is based on the relationships that exist between isoprenoid emissions and LUE as a result of the greater availability of photosynthetic reducing power for isoprenoid production under lower LUEs, that is under a higher excess of photosynthetically active radiation (PAR) that is not used for fixing carbon [12] , [21] , [22] and based on the fact that PRI is already widely tested as a good estimator of LUE at the leaf, canopy and ecosystem levels [23] , [24] , [25] , [27] . The better fit of LUE with percentages of isoprenoid emissions relative to the maximum than with absolute values ( Figs 2 , 3 ) warrants further efforts to develop the standardization of the signal for different species, ecosystems and conditions by gaining the necessary knowledge on the scaling physiological and structural processes involved. PRI is a remote sensing index that not only relates to the physiological modulation of the maximum emission rates but also provides assessment of the physiological and structural conditions themselves, thus providing a better fit of absolute emission rates with PRI ( Fig. 6 ) than for emissions relative to the maximum (data not shown). PRI accounted for part of the discrepancy between observed and model-estimated emissions both for isoprene and for monoterpenes ( Figs 7 , 8 ), thus supporting the potential for remote sensing to scale isoprenoid emissions. Because of that, the complementation of MEGAN estimations with PRI improved the predictions of the isoprenoid emissions ( Fig. 9 ). The significant part of the variation in emission rates captured by PRI is likely linked to the shifts in basal rates induced by different stress conditions [10] . PRI was defined at the leaf and canopy levels in the early 1990s in order to assess the efficiency of the use of absorbed photosynthetic active radiation by plants to photosynthesize (LUE) [23] , [24] . PRI calculated from the data provided by satellite imaging spectrometers is currently increasingly being applied at the ecosystem level [27] , [28] , [29] , [30] , [31] , [32] , [33] , [34] , [35] , opening up the possibility of significantly improving the accuracy of estimating spatial and temporal gross CO 2 uptake by vegetation using remote sensing [25] , [27] . Now, however, these results also create the possibility of using remote sensing to estimate isoprenoid emissions directly, based on a rough general relationship or at least indirectly through the improved modulation of the estimated emissions from factors of emission capacity ( E c ) using PRI. A comparison of the remote sensing of formaldehyde and PRI could validate this approach. PRI could thus substitute the serial empirical functions currently established in the emission models to better estimate current emissions. A complementary use of the remote sensing of formaldehyde and PRI could validate this approach. Adding information from PRI to the emission models might at least help to capture some spatial and temporal variability that the current models presently miss. PRI was originally defined to assess the short-term xanthophyll pigment changes that accompany plant stress [36] , [37] . These changes are linked to the dissipation of the excess absorbed energy that cannot be processed through photosynthesis, and which therefore reduces LUE [38] . This excess absorbed energy is available for isoprenoid production [12] , [21] , [22] . As these pigment changes translate into changes in reflectance at 531 nm, and as a reflectance of 570 nm is instead insensitive to short-term changes in these pigments, the PRI was defined as (R 531 −R 570 )/(R 531 +R 570 ), where R indicates reflectance and numbers indicate wavelength in nanometres [23] , [24] . Furthermore, the relationship with LUE is reinforced by the fact that PRI also measures the relative reflectance on either side of the green reflectance ‘hump’ (550 nm), that is, the reflectance in the blue region (chlorophyll and carotenoid absorption) of the spectrum relative to the reflectance in the red region (chlorophyll absorption only). Consequently, it also behaves as an index of chlorophyll:carotenoid ratios and therefore of the photosynthetic activities associated with their changes during leaf development, aging or stress in the longer term [39] , [40] , [41] ; it will probably also present an inverse relationship with isoprenoid emissions, as isoprenoids are also linked with carotenoids [20] . The isoprenoid–PRI relationships described here fit our current understanding of the physiological processes involved in isoprenoid emissions. Our study shows the potential of this PRI technique to validate the availability of photosynthetic reducing power as a factor involved in isoprenoid production and fits our hypothesis of isoprenoid emissions correlating with other more efficient energy quenching processes such as the xanthophyll cycle. Isoprenes and monoterpenes are synthesized via the plastidic 2- C -methyl-D-erythritol 4-phosphate pathway [42] , which is also the beginning of the synthesis route for essential metabolites, including the photoprotective compounds (carotenoids, tocopherol) [43] produced under stress conditions and lower LUE values. Demand for the various downstream products of the 2- C -methyl-D-erythritol 4-phosphate pathway can be a significant drain on photoassimilates, energy supply and reducing power [22] , [44] , [45] . The isoprenoid synthesis pathway consumes large amounts of photosynthetically formed adenosine triphosphate (ATP) and nicotinamide adenine dinucleotide phosphate (NADPH), and may thus serve as a ‘safety valve’ that is useful in avoiding over-reduction and photo-inhibition of the photosynthetic apparatus [12] , [21] , [22] , [46] . In fact, trade-offs between the attainment of optimal photosynthetic rates and volatile isoprenoids would appear to be inevitable when considering the overall allocation of carbon and energy supplies [12] , [21] , [22] . Isoprene and monoterpene emissions should thus be negatively correlated with LUE and with PRI. This is what we found here. Our results tend to confirm this hypothesis. PRI was negatively correlated with isoprenoid emissions that increased with rising irradiance and decreasing LUE. PRI was also effective in assessing isoprenoid emissions in senescing leaves but not in leaves of saplings suffering from drought conditions. This drought-related disturbance in the LUE–PRI relationship has already been found in the first studies using PRI to assess LUE under drought stress [23] , [36] . Isoprenoid emissions were negatively related to changes in LUE, both for isoprene in P. nigra and for monoterpenes in Q. ilex in response to irradiance, in each particular light growth environment ( Fig. 1 ). ATP and NADPH are needed in order to produce dimethylallyl diphosphate (DMAPP), the synthesis precursor of isoprene and monoterpenes [47] . There are more ‘excess’ electrons (and carbon chains) available for isoprene production in high than in low irradiance. Plants grown in full sunlight moreover develop higher capacities for the synthesis of isoprene and monoterpenes than do plants grown in the shade ( Fig. 1 ). When photosynthesis is electron transport-limited (in low light conditions), the shortfall of ATP and NADPH for CO 2 assimilation may cause a deficit in the reducing power available to transform carbohydrates into DMAPP. When photosynthesis is Rubisco-limited (in full light conditions), the plant may use a proportion of the ATP and NADPH excess (resulting from an excess of electrons produced by photochemical reactions) to reduce carbohydrates to DMAPP [12] , [21] , [22] , [47] and, as a result, isoprenoid emissions increase when light availability exceeds photosynthetic capacity. The fraction of the assimilated carbon allocated to isoprene production increases with increasing light intensity, even when photosynthesis is light-saturated [48] . Senescent leaves had slightly lower emission rates in our study and strong relationships with both LUE and PRI. The literature regarding isoprenoid emissions in ageing leaves is not very consistent: some studies suggest that the biochemical capacity to produce isoprene is unaffected by senescence, some others suggest that isoprene declines before photosynthesis, whereas some argue that measurable isoprene emission persists in senescing leaves even after the cessation of photosynthesis [12] . In poplars grown under conditions of elevated CO 2 , isoprene emission was sustained for longer periods in senescing leaves, whereas the decline in photosynthesis was accelerated [49] . Under these conditions, Tallis et al. [50] demonstrate an increased expression of genes involved in glycolysis, suggesting that phosphoenolpyruvic acid from glycolysis, translocated to the chloroplast, may provide the substrate for sustained isoprenoid emission in senescing leaves [51] . Under drought conditions, c i (internal CO 2 ) is reduced, as is photosynthetic carbon fixation ( Fig. 4 ) Although isoprenoid emissions are dependent on photosynthesis for the supply of energy (ATP), reducing power (NADPH) and carbon skeletons, several environmental and ontogenetic factors decouple the two processes. For instance, soil water deficits reduce photosynthetic carbon assimilation, whereas isoprene emissions can continue at a high level [52] . Light-dependent isoprene emission has been observed in leaves that have been severed at the stem and have ceased to photosynthesize [53] , [54] . At the leaf and canopy levels, there is an emerging consistency in the LUE–PRI relationship that suggests a functional convergence of biochemical, physiological and structural components affecting leaf, canopy and ecosystem carbon uptake efficiencies. The use of PRI as a proxy of LUE has extended exponentially in the last few years, both in natural and seminatural vegetation and in crops [27] . The results of these studies confirm an exponential relationship between LUE and PRI over a wide range of species and conditions, therefore suggesting that the relationship of isoprenoid emissions with PRI may also hold well when upscaled to the canopy and ecosystem scales. The high spectral resolution sensors on satellite platforms, such as the moderate resolution imaging spectroradiometer MODIS sensor on the TERRA and AQUA satellites, might therefore be used for global assessment of isoprenoid emissions. The results showed that the different sapling treatments with different environmental constraints and different LUE values present a different parameterization of their isoprenoid–PRI relationships, as happens with LUE–PRI exponential relationships [27] , [34] . PRI can be improved in the near future with standardization by species or biomes or environmental conditions, for example by comparison with different sensor angles or using other approaches in order to buffer the disturbing effects of geometry and structure of each type of species or ecosystem or environmental condition. However, in any case, although only approximate, there was a common exponential relationship between isoprenoid emissions and PRI, as there was for LUE–PRI relationships [27] ( Figs 2 , 4 ). Furthermore, even if no general isoprenoid emissions–PRI relationship can finally be established, PRI could at least be used as a modulator or scaling factor for the basal emission factors used for each species, biome or set of conditions ( Figs 1 , 5 , 9 ). The species- and ecosystem-specificity of BVOC emissions–PRI response curves creates a similar restriction to that of the current approach of using basal emission rates, but the use of PRI introduces a key improvement because PRI assesses emission rates actually, instead of assuming constant basal emission factors that in fact are very variable [9] , [10] . Satellite sensors such as MODIS can make suitable reflectivity measurements only once a day at a given location on the Earth in cloud free conditions. The PRI would thus suffer from an inherent clear sky bias, but it could be complemented with the use of remote sensing signals for HCHO that contain the underlying signature of BVOC emitted in both cloudy and clear sky conditions. These results therefore provide a challenging and exciting new way of potentially assessing isoprenoid emissions from terrestrial ecosystems, something which is essential for a more accurate quantification of global isoprenoid emissions and an understanding of their variability. PRI, as a proxy of isoprenoid emissions and LUE, can be used to complement the normalized difference vegetation index or other indices such as enhanced vegetation index, which are proxies of green biomass-fraction of absorbed PAR, in order to estimate canopy isoprenoid emission rates. There are other steps to take up before the generalization of PRI from the leaf level to the ecosystem and biospheric scales, and its global and operational use as an estimator of isoprenoid emissions. In brief, similar issues as those for PRI assessment of LUE at the ecosystem and biospheric scales can be encountered. These issues can be related to structural differences in the canopies, to varying ‘background effects’ (for example, soil colour, moisture, shadows, or the presence of other non-green landscape components), or to the different reflectance signals derived from illumination and variations in viewing angles [35] , [55] , [56] . Because of these issues, PRI may be more broadly applicable and portable across climatically and structurally different biome types when the differences in canopy structure are known [35] . However, several studies have found an emerging consistency in the relationship between PRI, LUE and ecosystem CO 2 uptake [27] , [28] , [29] , [30] , [31] , [32] , [33] , [34] , suggesting a surprising degree of ‘functional convergence’ in the biochemical, physiological and structural components affecting ecosystem carbon fluxes [57] , which can now be extended to isoprenoid emissions. In other words, ecosystem functioning possesses emergent properties that may allow us to explore their seemingly complex isoprenoid and photosynthetic behaviour effectively by using surprisingly simple optical sampling methods, such as the measurement of PRI or other remote sensing indices, algorithms and products that may emerge from the research effort in this area. Understanding the basis for this convergence and unearthing the ‘ecophysiological rules’ governing these responses each remain a primary goal of current ecophysiological research. Meanwhile, of importance for the pragmatic empirical remote sensing of isoprenoid emissions, PRI can assess the LUE of ecosystems, in particular from near-nadir satellite observations [34] ; with multiangle atmospheric correction [35] , [58] PRI also has the capacity to become an excellent tool in the continuous global monitoring of isoprenoid emissions, something that is essential in determining their chemical and climatic effects. The launching of a new image spectrometer, such as the NASA HyspIRI or the German EnMAP, will allow PRI to be calculated even at 30-m resolution: this offers great potential. The use of PRI will enable a better estimation of isoprenoid emissions, either through direct empirical estimates or through improved modelling, by modulating the emission factors for ecosystems and biomes rather than multiple complicated climatic, historical, and structural factors. Plant material and experimental setup We used 4-year-old potted P. nigra L. and Q. ilex L. plants grown in a nursery (Tres Turons S.C.P., Castellar del Vallès, Catalonia, Spain), maintained under Mediterranean ambient conditions outdoors (five saplings of each species grown under sunny conditions and five saplings grown under shade conditions). They were grown in 15-L pots with a substrate composed of peat and sand (2:1). To widen the range of tested LUE conditions, an additional plant treatment was established. Irrigation was withheld from these saplings grown under sunny and shaded conditions and, after 10–15 days, they were measured again (droughted plants). In order to further widen the range of tested LUE conditions for the control, P. nigra saplings grown in both sunny and shaded conditions were also measured in November when the leaves were senescing (senescing leaves). Three plants were measured per treatment. For each measurement, a small leaf chamber was clamped to a leaf. This leaf cuvette was part of a LCpro+ photosynthesis system (ADC BioScientific, Herts, England), which recorded photosynthesis (net CO 2 uptake), stomatal conductance, air humidity and temperature data, while controlling light and the flow of air entering the leaf cuvette. A light-response curve was programmed into the leaf chamber, ranging from 0 to 2,500 μmol m –2 s –1 of PAR ( Fig. 4 ); measurements were made continuously for 45 min at each light intensity and at a constant temperature of 30 °C. Plant reflectance measurements The reflectance of the clamped leaf was simultaneously measured with a UniSpec Spectral Analysis System/Reflectometer (PP Systems, Haverhill, MA, USA) operated using a palmtop PC. Fifty scans were integrated (integration time 10 ms) per sample. Reflectance measurements were preceded by a dark scan and compared with reflectance measurements from a Spectralon (Labsphere, North Sutton, NH, USA) white standard in order to obtain the reflectance values. PRI was calculated as (R531−R570)/(R531+R570), where Rn is the reflectance of the leaf at n nm [24] . CO 2 and BVOC exchange measurements Foliar CO 2 and H 2 O exchanges were measured with the LCpro+ Photosynthesis System (ADC BioScientific). LUE was here calculated as the ratio between the net photosynthetic rates and incident PAR. In order to determine and quantify BVOC exchange, flow meter were used to monitor the air exiting the leaf chamber, which was then analysed using proton transfer reaction–mass spectrometry (PTR–MS; Ionicon Analytik, Innsbruck, Austria). At alternative intervals, the output air flowing from the leaf chamber was also sampled using stainless steel tubes filled with terpene adsorbents, and thereafter analysed by thermal desorption and gas chromatography–mass spectrometry (GC–MS). The difference between the concentration of isoprenoids passing through the chamber clamped to a leaf and the chamber with no leaf, together with the flow rates, were used to calculate the foliar isoprenoid exchange. The tubing used to connect the leaf chamber with the PTR–MS system (50 cm long and 2 mm internal diameter) was made of Teflon. The system used was always the same for all measurements. The PTR–MS technique PTR–MS is based on chemical ionization, specifically non-dissociative proton transfer from H 3 O + ions to most of the common BVOCs, and has been fully described elsewhere [59] . In our experiment, the PTR–MS drift tube was operated at 2.1 mbar and 50 °C, with an E/N (electric field/molecule number density) of around 130 Td (townsend) (1 Td=10 –17 V cm 2 ). The primary ion signal (H 3 O + ) was maintained at approximately 6 × 10 6 counts per second. The instrument was calibrated using an aromatic mix standard gas (TO-14A, Restek, Bellefonte, PA, USA) and isoprene and monoterpene standard gas (Abello Linde SA, Barcelona). Terpene sampling and analysis by GC–MS Exhaust air from the chambers was pumped through a stainless steel tube (8 cm long and 0.3 cm internal diameter), filled manually with the terpene adsorbents Carbopack B, Carboxen 1,003 and Carbopack Y (Supelco, Bellefonte, Pennsylvania), and separated by plugs of quartz wool. Samples were taken using a Qmax air sampling pump (Supelco, Bellefonte, PE, USA). For more details see Peñuelas et al. [60] The sampling time was 10 min, and the flow varied between 470 and 500 ml min −1 depending on the glass tube adsorbent and quartz wool packing. Glass tubes were stored at −28 °C until the analysis. Terpene analyses were performed using a GC–MS system (Hewlett Packard HP59822B, Palo Alto, CA, USA). The monoterpenes trapped on the tubes were processed with an automatic sample processor (Combi PAL, FOCUS-ATAS GL International BV 5500 AA Veldhoven, The Netherlands) and desorbed, using an OPTIC3 injector (ATAS GL International BV 5500 AA Veldhoven, The Netherlands), into a 30 × 0.25 × 0.25 mm film capillary column (SPB TM-5 Fused Silica Capillary column; Supelco, Bellefonte, PE, USA). The injector temperature (60 °C) was increased at 16 °C s −1 to 300 °C. The injected sample was cryofocused at −20 °C for 2 min. After this time, the cryotrap was heated rapidly to 250 °C. Helium flow was 0.7 ml min −1 . Total run time was 23 min and the solvent delay was 4 min. After the sample injection, the initial temperature (40 °C) was increased at 30 °C min −1 up to 60 °C, and thereafter at 10 °C min −1 up to 150 °C. This temperature was maintained for 3 min, and thereafter increased at 70 °C min −1 up to 250 °C, and maintained at this temperature for another 5 min. Helium flow was 1 ml min −1 . Monoterpenes were identified by comparing the retention times with standards from Fluka (Buchs, Switzerland), and the fractionation mass spectra with standards, spectra derived from the literature and the GCD Chemstation G1074A HP and the mass spectra library wiley7n. Terpene concentrations were determined from calibration curves. The calibration curves for common monoterpenes, a-pinene, D 3 -carene, b-pinene, b-myrcene, p -cymene, limonene and sabinene, and common sesquiterpenes such as a-humulene, were determined once every five analyses using four different terpene concentrations. The calibration curves were always highly significant ( r 2 >0.99 for the relationships between the signal and terpene concentrations). Data treatment Linear and non-linear curves were fitted using Sigmaplot and statistical tests with Statistica 6.0 software (StatSoft, Tulsa, OK, USA). We used R (RKWard Version 0.6.1) [61] to develop empirical models based on the exponential and linear relationships between emissions and PRI found as a result of repeated random sub-sampling of two out of three replicates for each growth condition as the training set for estimating the isoprenoid emission rates. The estimated values were then tested against the values of the remaining randomly selected third set of replicates. This procedure was repeated 1,000 times. Emissions were also estimated with MEGAN model algorithms [3] , and with empirical models using MEGAN algorithms complemented with PRI. How to cite this article: Peñuelas, J. et al. Photochemical reflectance index as an indirect estimator of foliar isoprenoid emissions at the ecosystem level. Nat. Commun. 4:2604 doi: 10.1038/ncomms3604 (2013).